HSV-1 exploits the innate immune scavenger receptor MARCO to enhance epithelial adsorption and infection Herpes simplex virus type 1 is an important epithelial pathogen and has the potential for significant morbidity in humans. Here we demonstrate that a cell surface scavenger receptor, macrophage receptor with collagenous structure (MARCO), previously thought to enhance antiviral defense by enabling nucleic acid recognition, is usurped by herpes simplex virus type 1 and functions together with heparan sulphate proteoglycans to mediate adsorption to epithelial cells. Ligands of MARCO dramatically inhibit herpes simplex virus type 1 adsorption and infection of human keratinocytes and protect mice against infection. Herpes simplex virus type 1 glycoprotein C closely co-localizes with MARCO at the cell surface, and glycoprotein C binds directly to purified MARCO with high affinity. Increasing MARCO expression enhances herpes simplex virus type 1 infection while MARCO −/− mice have reduced susceptibility to infection by herpes simplex virus type 1. These findings demonstrate that herpes simplex virus type 1 binds to MARCO to enhance its capacity for disease, and suggests a new therapeutic target to alter pathogenicity of herpes simplex virus type 1 in skin infection. Herpes simplex virus type 1 (HSV-1) infections are a frequent occurrence and have the potential to develop into life-threatening disease in immunocompromised individuals. Primary infection typically begins in the skin and mucocutaneous regions by targeting keratinocytes, the most abundant cell type in these tissues. If infection is not controlled, HSV-1 can spread to other target organs including the central nervous system (CNS). Despite advances in antiviral therapies that have reduced HSV morbidity and mortality, it remains of considerable interest to understand in greater detail the elements contributing to HSV-1 virulence. Towards this end, a more detailed analysis of the host elements that are used by the virus to promote infection and the local elements of the mucocutaneous defense system that act to resist HSV-1 infection is needed. HSV-1 initiates disease by repurposing host-derived molecules to enhance its virulence. The first step in this process is adsorption of the virus to the cell surface. Heparan sulphate proteoglycans (HSPGs) were the only known molecules on the host cell responsible for this process [1] . Interestingly, HSV-1 and HSV-2 both bind to HSPGs yet recognize different structural features of heparan sulphate, thus showing that there is some degree of specificity to this interaction [2] . Glycoprotein C (gC) is the major HSV-1 glycoprotein that binds to HSPGs [3] , [4] , but glycoprotein B (gB) also contributes to HSPG adsorption, and this is particularly important in the absence of gC [5] . The HSPGs Syndecan-1 and Syndecan-4 are highly expressed by keratinocytes [6] and may serve as adsorption receptors for HSV-1, however, studies have not addressed which specific receptors expressed by keratinocytes are most vital for adsorption. Membrane fusion events follow adsorption and additionally involve interactions of HSV-1 glycoprotein D (gD) and gB with the cell surface. Multiple cell surface targets have been identified for viral entry including for gD: 3-O-sulphated heparan sulphate [7] , tumour necrosis factor receptor superfamily member 14 (commonly known as herpesvirus entry mediator) [8] or poliovirus receptor-related protein 1 (commonly known as Nectin-1) (ref. 9 ), and for gB: paired immunoglobulin-like type 2 receptor alpha [10] or myosin-9 (also known as non-muscle myosin IIa) [11] . To mount an effective antiviral response, cells must recognize the virus and initiate an appropriate immune response. Several types of innate immune receptors have been associated with the capacity to detect HSV infection [12] . Class A scavenger receptors are an important element in this innate immune detection process as they bind to extracellular viral double-stranded RNA (dsRNA) at the cell surface to mediate dsRNA uptake and to enable this dsRNA to interact with TLR3 in the endosome [13] , [14] , [15] , [16] , [17] . Failures of this TLR3-dependent innate immune recognition pathway can have serious consequences. For example, human patients with genetic defects in TLR3 (ref. 18 ), and other proteins involved in mediating the TLR3-dependent response to dsRNA [19] , [20] , [21] , are predisposed to herpes simplex encephalitis, a severe, disseminated infection of the CNS, and TLR3 deficiency in mice renders astrocytes more susceptible to HSV infection and leads to HSV-mediated disease in the CNS [22] . It is hypothesized that TLR3 is important for recognition of a DNA virus such as HSV-1 because virtually all viruses produce dsRNA during replication [23] , and this dsRNA is released into extracellular space following lysis of infected cells [24] . Thus, cells expressing TLR3 have the ability to defend against HSV-1 by using this receptor to respond to dsRNA, and this appears to be particularly crucial to innate antiviral defense in the CNS. Here we present the unexpected discovery that instead of contributing to host defense, the class A scavenger receptor macrophage receptor with collagenous structure (MARCO) is exploited by HSV-1 to promote cell surface adsorption and infection in the skin. Scavenger receptor ligands inhibit HSV-1 infection Surface epithelial cells are the initial target for viral entry and can activate a potent innate immune response through TLR3 (refs 25 , 26 , 27 , 28 ). Activation of TLR3 increases pro-inflammatory cytokines, antimicrobial peptides and interferons (IFNs) in skin and other tissues [29] , [30] , [31] , and has been frequently linked with cutaneous immune and antiviral responses [25] , [32] , [33] . We first sought to determine whether activation of TLR3 could enable keratinocytes to directly defend themselves against HSV-1 by treating cells with Poly(I:C), a synthetic dsRNA [25] , [26] , [27] , [28] . Poly(I:C) treatment resulted in inhibition of HSV-1 infection as assessed by measuring levels of HSV-1 gD messenger RNA ( Fig. 1a ). However, TLR3 activation appeared to be dispensible for this protection against infection as treatment with Poly(I), a single-stranded RNA component of Poly(I:C) that does not activate TLR3, conferred protection against HSV-1 similar to that seen with Poly(I:C) ( Fig. 1a ). Poly(I) and Poly(C) were not able to increase expression of IL-6, IL-8, IFN-β and human beta-defensin 2 (hBD-2), four genes that were significantly increased by Poly(I:C) stimulation of normal human epidermal keratinocytes (NHEK) ( Fig. 1b ). Furthermore, inhibition of IFN-β production by methyl thioadenosine [34] , a signal transducer and activator of transcription 1 inhibitor, did not alter the capacity of Poly(I:C) to reduce HSV-1 gD expression ( Supplementary Fig. S1a,b ). These results indicated that although IFN-β has well-characterized antiviral effects [35] , [36] , it was not responsible for protection against HSV-1 infection by Poly(I:C) under these conditions. We confirmed these results by utilizing chloroquine (CQ) to more directly examine the effect of TLR3 inhibition on the ability of Poly(I:C) to protect against HSV-1 infection, as CQ is known to be a potent inhibitor of endosomal acidification and TLR3 activation [16] . As expected, pretreatment with CQ inhibited the capacity of Poly(I:C) to stimulate expression of IL-6 and IFN-β, thus confirming that TLR3 activation was inhibited ( Supplementary Fig. S1c ). However, despite inhibition of cytokine and interferon responses, CQ did not reduce the capacity of Poly(I:C) to protect against HSV-1 infection ( Supplementary Fig. S1d ), further showing that cellular activation mediated by TLR3 was not required for the protective effects of Poly(I:C). Therefore, as Poly(I) was capable of inhibiting HSV-1 infection, but Poly(C) was not, we considered alternate explanations that could account for the antiviral activity of both Poly(I) and Poly(I:C). 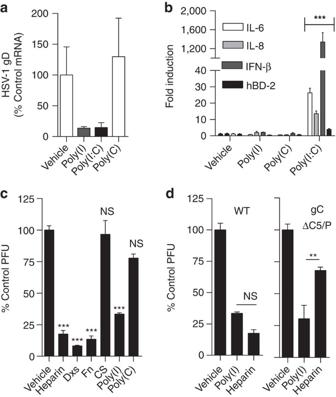Figure 1: Scavenger receptor ligands inhibit HSV-1 infection of keratinocytes. (a) HaCats were treated with 100 μg ml−1Poly(I:C), or 50 μg ml−1of Poly(I) or Poly(C) 20 min before the addition of HSV-1 at a multiplicity of infection (MOI) of 0.01. Cells were incubated for 5.5 h before quantification of HSV-1 messenger RNA by quantitative PCR (qPCR). (b) NHEK were treated with 10 μg ml−1Poly(I), Poly(C) and Poly(I:C) for 3 h before qPCR analysis of gene expression. (c) NHEK were treated with 10 μg ml−1of the indicated compounds for 20 min before the addition of HSV-1 at an MOI of 0.0005. Plaque forming units (PFU) were quantified 48 h after infection. (d) NHEK were treated with 10 μg ml−1Poly(I) or heparin 20 min before infection with WT HSV-1 at an MOI of 0.0005 or an equivalent amount of HSV-1 gCΔC5/P (HSV-1 possessing gC with a deletion of the heparin-binding domain, amino acids 33–123) viral particles. PFU were quantified 48 h after infection. PFU are displayed as relative % compared with untreated cells for each virus. NS, not significant. (a–d) all data are means±s.e.m,n=3 from representative experiments repeated at least two times. One-way analysis of variance (ANOVA) with Tukey post-tests were used for statistical analysis, **P<0.01; ***P<0.001. (b,c)P-values were derived from comparisons to vehicle-treated samples. Figure 1: Scavenger receptor ligands inhibit HSV-1 infection of keratinocytes. ( a ) HaCats were treated with 100 μg ml −1 Poly(I:C), or 50 μg ml −1 of Poly(I) or Poly(C) 20 min before the addition of HSV-1 at a multiplicity of infection (MOI) of 0.01. Cells were incubated for 5.5 h before quantification of HSV-1 messenger RNA by quantitative PCR (qPCR). ( b ) NHEK were treated with 10 μg ml −1 Poly(I), Poly(C) and Poly(I:C) for 3 h before qPCR analysis of gene expression. ( c ) NHEK were treated with 10 μg ml −1 of the indicated compounds for 20 min before the addition of HSV-1 at an MOI of 0.0005. Plaque forming units (PFU) were quantified 48 h after infection. ( d ) NHEK were treated with 10 μg ml −1 Poly(I) or heparin 20 min before infection with WT HSV-1 at an MOI of 0.0005 or an equivalent amount of HSV-1 gCΔC5/P (HSV-1 possessing gC with a deletion of the heparin-binding domain, amino acids 33–123) viral particles. PFU were quantified 48 h after infection. PFU are displayed as relative % compared with untreated cells for each virus. NS, not significant. ( a – d ) all data are means±s.e.m, n =3 from representative experiments repeated at least two times. One-way analysis of variance (ANOVA) with Tukey post-tests were used for statistical analysis, ** P <0.01; *** P <0.001. ( b , c ) P -values were derived from comparisons to vehicle-treated samples. Full size image Both Poly(I) and Poly(I:C) are ligands for class A scavenger receptors, a family of cell surface molecules required for dsRNA uptake before cell activation [13] , [14] , [15] , [37] . Poly(C), which did not protect against HSV-1, is not a ligand for class A scavenger receptors. Therefore, we next hypothesized that the capacity to inhibit infection was related to the ability to bind scavenger receptors. To test this hypothesis, we examined additional scavenger receptors ligands: Fucoidan (Fn) and dextran sulphate (Dxs). These were chosen as they also bind scavenger receptors [37] but are structurally distinct from the polynucleotides. The capacity of Dxs, Fn and Poly(I) to bind scavenger receptors was confirmed by showing their ability to block Poly(I:C) stimulation of cytokine release ( Supplementary Fig. S1e,f ). Chondroitin sulphate (CS) was used as a control for Dxs and Fn as it is another sulphated polysaccharide, but like Poly(C) it cannot bind scavenger receptors, and had no effect on the capacity of Poly (I:C) to function ( Supplementary Fig. S1f ). Diverse molecules that share the capacity to bind scavenger receptors (Poly(I), Dxs and Fn) all reduced HSV-1 plaque formation, but similar control molecules CS and Poly(C) did not ( Fig. 1c ). However, heparin also inhibited HSV-1 infection in NHEK ( Fig. 1c ). This effect was previously known and thought to occur by inhibiting the interaction of HSV-1 with cell surface HSPGs [1] . Therefore, we next examined if scavenger receptor ligands might act by interference with adsorption to HSPGs. To first test this, we compared the capacity of Poly(I) and heparin to inhibit infection by a mutant form of HSV-1 that has a truncated gC lacking amino acids 33–123, the C5/P domain (gCΔC5/P) predominantly responsible for heparin binding [4] , [38] . As expected, heparin treatment inhibited infection of wild-type (WT) virus but had a less potent inhibitory effect on the mutant virus lacking this heparin-binding domain ( Fig. 1d ). However, Poly(I) similarly inhibited infection of both the WT virus and the gCΔC5/P mutant. These results, together with our previous findings, led us to hypothesize that HSV-1 infection of keratinocytes involves a previously unsuspected interaction with both a scavenger receptor and HSPGs acting together to mediate adsorption to keratinocytes. Scavenger receptor ligands inhibit HSV-1 and gC adsorption We next tested the action of scavenger receptors ligands in the initial adsorption of HSV-1 to cell surfaces. Poly(I) prevented adsorption of whole HSV-1 viral particles to keratinocytes in a dose-dependent manner, while increasing doses of Poly(C) had no effect ( Fig. 2a ). As adsorption of HSV-1 to the cell surface is primarily mediated by the viral glycoprotein gC [3] , [4] , we next analysed the effects of Poly(I) on binding of this purified protein to the keratinocyte surface. The association of purified gC with NHEK was inhibited by Poly(I), but not Poly(C) ( Fig. 2b ). Furthermore, as predicted from prior work, heparin blocked the association of gC with cell surface HSPGs [1] ( Fig. 2b ). However, Poly(I) inhibited binding of gC by a different mechanism than heparin because Poly(I) could not displace gC from a heparin column ( Fig. 2c ). In contrast, gC was easily displaced from heparin by sodium chloride concentrations below 1.0 M ( Fig. 2d ), suggesting a relatively weak ionic interaction. These results show that HSV-1 gC binds to keratinocytes by both heparan sulphate-dependent and heparan sulphate-independent mechanisms, and Poly(I) acted on the heparan sulphate-independent binding event. 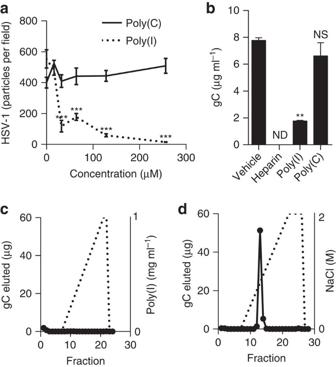Figure 2: Effect of scavenger receptor ligands on adsorption of HSV-1 and purified gC. (a) HaCat keratinocytes were incubated with HSV-1 at a multiplicity of infection of 100 at 4 °C with the indicated concentrations of Poly(I) and Poly(C). Bound HSV-1 was visualized by fluorescence microscopy. Five images of bound HSV-1 per concentration were captured and the number of HSV-1 particles quantified using ImageJ. Each image contained 15–20 cells. Error bars indicate s.e.m. Two-way analysis of variance (ANOVA) with bonferroni post-tests was used to compare the effect of Poly(I) to Poly(C).n=5, ***P<0.001. (b) purified gC was incubated with NHEK in the presence of 100 μg ml−1heparin, Poly(I) or Poly(C) at 4 °C. Unbound gC was removed by multiple wash steps, then cells were fixed and bound gC was detected and quantified using an on-cell western assay. Error bars indicate s.e.m. One-way ANOVA with Tukey post-tests were used for statistical analysis with comparisons made to vehicle-treated cells,n=2, **P<0.01. ND, not detectable, NS, not significant. (c,d) One-hundred micrograms of purified gC was bound to a Heparin column, and eluted with a linear gradient (broken line) of Poly(I) (c), or NaCl (d). Eluted gC was quantified from 1 ml fractions by dot blot and plotted as solid black circles representing each individual fraction connected by a solid line. Figure 2: Effect of scavenger receptor ligands on adsorption of HSV-1 and purified gC. ( a ) HaCat keratinocytes were incubated with HSV-1 at a multiplicity of infection of 100 at 4 °C with the indicated concentrations of Poly(I) and Poly(C). Bound HSV-1 was visualized by fluorescence microscopy. Five images of bound HSV-1 per concentration were captured and the number of HSV-1 particles quantified using ImageJ. Each image contained 15–20 cells. Error bars indicate s.e.m. Two-way analysis of variance (ANOVA) with bonferroni post-tests was used to compare the effect of Poly(I) to Poly(C). n =5, *** P <0.001. ( b ) purified gC was incubated with NHEK in the presence of 100 μg ml −1 heparin, Poly(I) or Poly(C) at 4 °C. Unbound gC was removed by multiple wash steps, then cells were fixed and bound gC was detected and quantified using an on-cell western assay. Error bars indicate s.e.m. One-way ANOVA with Tukey post-tests were used for statistical analysis with comparisons made to vehicle-treated cells, n =2, ** P <0.01. ND, not detectable, NS, not significant. ( c , d ) One-hundred micrograms of purified gC was bound to a Heparin column, and eluted with a linear gradient (broken line) of Poly(I) ( c ), or NaCl ( d ). Eluted gC was quantified from 1 ml fractions by dot blot and plotted as solid black circles representing each individual fraction connected by a solid line. Full size image MARCO co-localizes with HSV-1 virions and purified gC We next sought to identify a specific scavenger receptor on keratinocytes that could associate with HSV-1 gC. Analysis of NHEK determined that these cells express multiple scavenger receptors including MARCO, OLR1 and SCARA3 ( Supplementary Fig. S2 ). These receptors can all bind Poly(I) (refs 39 , 40 , 41 , 42 ), and thus we sought to determine if these receptors could co-localize with HSV-1 bound to the cell surface. To specifically measure co-localization with HSV-1 gC, we employed a proximity ligation assay (PLA) that is designed to generate a fluorescent signal only when the antigens tested reside within less than ~40 nm from one another. Assays were performed by maintaining cells at 4 °C to inhibit glycoprotein uptake and viral entry, and comparisons were made between co-localization of HSV-1 gC with MARCO, syndecan-1, OLR1 and SCARA3. Syndecan-1, an HSPG previously linked to HSV-1 infection [43] , [44] , generated a positive PLA signal in the presence of gC ( Fig. 3b ), confirming that this HSPG co-localized with gC. MARCO also generated a strong positive PLA signal ( Fig. 3a ), indicating that MARCO and gC are residing on the surface of the cells in close physical proximity in the absence of other viral components. OLR1 and SCARA3, although abundantly expressed on the cell surface ( Supplementary Fig. S2 ), did not co-localize with HSV-1 gC ( Fig. 3c ). Similarly, when whole virions were added instead of glycoprotein, a strong PLA signal was generated with either MARCO or syndecan-1, but not OLR1 or SCARA3 ( Supplementary Fig. S3 ), confirming the selective, close co-localization of MARCO and syndecan-1 with HSV-1 gC. 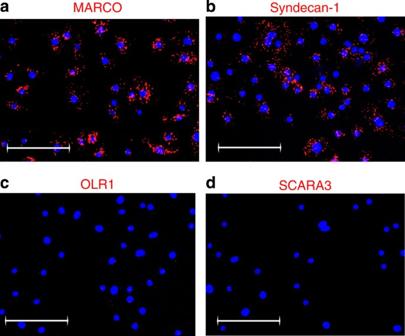Figure 3: MARCO co-localizes with HSV-1 gC on the keratinocyte cell surface. NHEK were incubated in the presence of purified HSV-1 gC for 2 h at 4 °C to allow binding of the glycoprotein to the cell surface. Unbound gC was removed by multiple wash steps before cells were fixed and incubated with both a mouse monoclonal antibody targeting HSV-1 gC, and rabbit polyclonal antibodies targeting MARCO (a), syndecan-1 (b), OLR1 (c) or SCARA3 (d). Physical proximity of MARCO, syndecan-1, OLR1 or SCARA3 to HSV-1 gC bound to the cell surface was determined using a fluorescence-based PLA that produces a red fluorescent signal only when the antigens recognized by the antibodies utilized in the assay reside within <40 nm of each other. Nuclei (blue) are stained with Hoescht. Scale bar, 100 μm. All data are from representative experiments repeated 2–4 times. Figure 3: MARCO co-localizes with HSV-1 gC on the keratinocyte cell surface. NHEK were incubated in the presence of purified HSV-1 gC for 2 h at 4 °C to allow binding of the glycoprotein to the cell surface. Unbound gC was removed by multiple wash steps before cells were fixed and incubated with both a mouse monoclonal antibody targeting HSV-1 gC, and rabbit polyclonal antibodies targeting MARCO ( a ), syndecan-1 ( b ), OLR1 ( c ) or SCARA3 ( d ). Physical proximity of MARCO, syndecan-1, OLR1 or SCARA3 to HSV-1 gC bound to the cell surface was determined using a fluorescence-based PLA that produces a red fluorescent signal only when the antigens recognized by the antibodies utilized in the assay reside within <40 nm of each other. Nuclei (blue) are stained with Hoescht. Scale bar, 100 μm. All data are from representative experiments repeated 2–4 times. Full size image MARCO directly binds to HSV-1 gC The experiments described above implied that MARCO can interact directly with HSV-1 gC. We next used purified MARCO to verify that gC can bind to this protein in the absence of other cellular receptors and to determine the affinity of this interaction. gC bound at nM concentrations to MARCO, to saturation, and with association plots suggesting single order specific binding ( Fig. 4a ). This effect was specific to gC and MARCO, as another viral glycoprotein, gB, did not bind to MARCO ( Fig. 4c ), and gC did not bind to an alternative scavenger receptor, OLR1 ( Fig. 4d ). Notably, the interaction between MARCO and gC had a K D of 7.7 × 10 −10 nM, a stronger affinity than that reported previously between gC and heparan sulphate or heparin ( K D values of 1.3 × 10 −8 nM and 1 × 10 −7 nM, respectively, obtained by surface plasmon resonance) [38] . 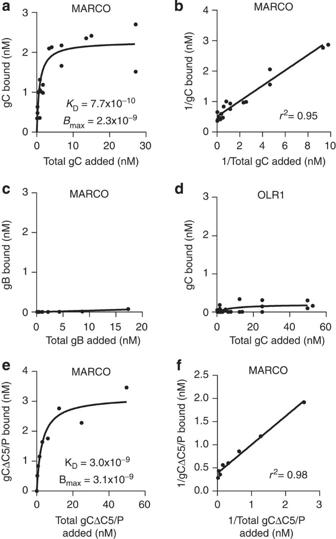Figure 4: MARCO binds directly to HSV-1 gC. Plate-bound purified MARCO protein was incubated with increasing concentrations of purified gC (a), gB (c) or gCΔC5/P (gC with a deletion of the heparin-binding domain, amino acids 33–123) (e). gC, gB and gCΔC5/P remaining bound after multiple wash steps was detected and quantified by ELISA. The dissociation constant (KD) and the maximum number of receptor-binding sites (Bmax) were determined using nonlinear regression with background subtracted using Graphpad Prism. Inbandf, data inaande, respectively, were transformed to create double-reciprocal plots to show linear-binding kinetics. (d) Plate-bound recombinant OLR 1 was incubated with purified gC. gC remaining bound after washing was detected and quantified by ELISA. (a–f) All individual replicate values plotted with offset overlapping points. All data are from representative experiments repeated at least two times. Figure 4: MARCO binds directly to HSV-1 gC. Plate-bound purified MARCO protein was incubated with increasing concentrations of purified gC ( a ), gB ( c ) or gCΔC5/P (gC with a deletion of the heparin-binding domain, amino acids 33–123) ( e ). gC, gB and gCΔC5/P remaining bound after multiple wash steps was detected and quantified by ELISA. The dissociation constant ( K D ) and the maximum number of receptor-binding sites ( B max ) were determined using nonlinear regression with background subtracted using Graphpad Prism. In b and f , data in a and e , respectively, were transformed to create double-reciprocal plots to show linear-binding kinetics. ( d ) Plate-bound recombinant OLR 1 was incubated with purified gC. gC remaining bound after washing was detected and quantified by ELISA. ( a – f ) All individual replicate values plotted with offset overlapping points. All data are from representative experiments repeated at least two times. Full size image Further evidence that HSV-1 gC adsorption to scavenger receptors is independent of adsorption to HSPG was seen by analysis of binding to gC lacking the heparin-binding (C5/P) domain (amino acids 33–123). This truncated form of gC binds heparin with ~42-fold lower affinity than the intact form of gC [38] but still bound to MARCO with relatively high affinity ( Fig. 4e ). The capacity of gC lacking the C5/P domain to bind to MARCO was consistent with our earlier finding that the infectivity of HSV-1 harbouring this mutated gC was strongly inhibited by Poly(I), while heparin had a less potent inhibitory effect compared with its capacity to inhibit infection by WT virus ( Fig. 1f ). HSV-1 infection correlates with MARCO expression To confirm the functional significance of the interaction of HSV-1 gC and MARCO, we next generated a HaCat keratinocyte cell line that stably overexpressed human MARCO. MARCO overexpressing cells expressed ~threefold more MARCO protein than control cells ( Fig. 5a , and Supplementary Fig. S4 ). Keratinocytes overexpressing MARCO were more susceptible to infection than a control cell line ( Fig. 5c ), demonstrating that increasing the expression of MARCO resulted in increased infection by HSV-1. Furthermore, the presence of gC was essential for this enhancement of infection, as a mutant virus lacking gC exhibited comparable levels of infection in control and MARCO overexpressing cells ( Fig. 5c ). 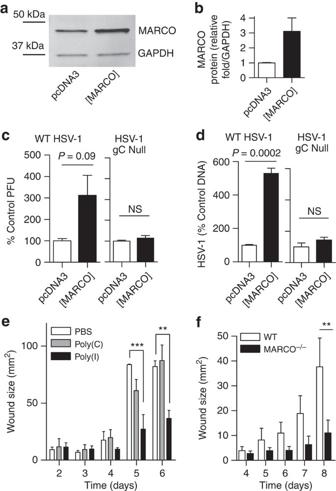Figure 5: HSV-1 infection correlates with MARCO expression in cells and in mice and is reduced by Poly(I). (a–d) HaCat cells were transfected with a control plasmid, pcDNA3 or a pcDNA3-backbone plasmid with the human MARCO gene inserted (labelled as [MARCO] on graphs) and selected with G418 to enable stable expression. MARCO and GAPDH protein levels were visualized in the same sample of 20 μg total protein using two-colour western blot (a). The image inais from one representative western blot of two blots, and the image of the full-length blot is presented inSupplementary Fig. S4. MARCO protein levels relative to GAPDH were quantified using Licor Odyssey software (b),n=2, error bars indicate the s.e.m. (c,d) pcDNA3 and [MARCO] cells were infected with WT or HSV-1 gC null (HSV-1 lacking gC) at a multiplicity of infection (MOI) of 0.0005. Plaque forming units (PFU) were quantified 48 h after infection (c) and viral DNA was quantified 24 h after infection (d). (c,d) Comparisons between pcDNA3 and [MARCO] cells were made using two-tailedT-tests,n=3. Error bars indicate the s.e.m. Data presented are from one representative experiment of at least two independent experiments. (e) Sixteen-week-old female mice were immunocompromised with cyclophosphamide before infection with HSV-1. Mice were injected subcutaneously with PBS, or 125 μg Poly(C) or Poly(I) twice daily at the site of infection beginning the first day of infection. Photographs were taken once daily beginning the first day post-infection. Lesions were quantified using ImageJ. Error bars indicate the s.e.m. Two-way analysis of variance (ANOVA) with bonferroni post-tests was used to compare wound sizes in Poly(I) and Poly(C)-treated mice to PBS-treated mice,n=4, **P<0.01; ***P<0.001. (f) Eleven-week-old sex-matched WT and MARCO−/−mice were immunocompromised with cyclophosphamide before infection with HSV-1. Mice were photographed daily until 8 days post-infection when WT mice began to exhibit symptoms of systemic and neurological infection, necessitating euthanasia. Lesion formation was quantified using ImageJ. Error bars indicate the s.e.m. Two-way ANOVA with bonferroni post-tests was used to compare wound sizes in WT and MARCO mice,n=5; **P<0.01. Data presented are from one representative experiment of two independent experiments. Figure 5: HSV-1 infection correlates with MARCO expression in cells and in mice and is reduced by Poly(I). ( a – d ) HaCat cells were transfected with a control plasmid, pcDNA3 or a pcDNA3-backbone plasmid with the human MARCO gene inserted (labelled as [MARCO] on graphs) and selected with G418 to enable stable expression. MARCO and GAPDH protein levels were visualized in the same sample of 20 μg total protein using two-colour western blot ( a ). The image in a is from one representative western blot of two blots, and the image of the full-length blot is presented in Supplementary Fig. S4 . MARCO protein levels relative to GAPDH were quantified using Licor Odyssey software ( b ), n =2, error bars indicate the s.e.m. ( c , d ) pcDNA3 and [MARCO] cells were infected with WT or HSV-1 gC null (HSV-1 lacking gC) at a multiplicity of infection (MOI) of 0.0005. Plaque forming units (PFU) were quantified 48 h after infection ( c ) and viral DNA was quantified 24 h after infection ( d ). ( c , d ) Comparisons between pcDNA3 and [MARCO] cells were made using two-tailed T -tests, n =3. Error bars indicate the s.e.m. Data presented are from one representative experiment of at least two independent experiments. ( e ) Sixteen-week-old female mice were immunocompromised with cyclophosphamide before infection with HSV-1. Mice were injected subcutaneously with PBS, or 125 μg Poly(C) or Poly(I) twice daily at the site of infection beginning the first day of infection. Photographs were taken once daily beginning the first day post-infection. Lesions were quantified using ImageJ. Error bars indicate the s.e.m. Two-way analysis of variance (ANOVA) with bonferroni post-tests was used to compare wound sizes in Poly(I) and Poly(C)-treated mice to PBS-treated mice, n =4, ** P <0.01; *** P <0.001. ( f ) Eleven-week-old sex-matched WT and MARCO −/− mice were immunocompromised with cyclophosphamide before infection with HSV-1. Mice were photographed daily until 8 days post-infection when WT mice began to exhibit symptoms of systemic and neurological infection, necessitating euthanasia. Lesion formation was quantified using ImageJ. Error bars indicate the s.e.m. Two-way ANOVA with bonferroni post-tests was used to compare wound sizes in WT and MARCO mice, n =5; ** P <0.01. Data presented are from one representative experiment of two independent experiments. Full size image Next, to test the relevance of disruption of scavenger receptors using an in vivo system, we employed a model of severe cutaneous HSV-1 infection and tested the capacity of Poly(I) to prevent HSV-1-mediated disease. Mice were immunocompromised by prior systemic cyclophosphamide treatment [45] , then infected with HSV-1 in the skin. Mice were treated locally with PBS, Poly(C) or Poly(I). Control mice treated with PBS or Poly(C) developed large necrotic skin lesions, but Poly(I) treatment significantly inhibited cutaneous lesion development ( Fig. 5e ). Finally, to confirm the role of MARCO in this in vivo model and demonstrate the functional relevance of the interaction of HSV-1 and MARCO, we compared infection in WT and MARCO −/− mice. Skin lesions in WT mice were larger than those seen in MARCO −/− mice, a difference that persisted and increased over the course of the experiment. By day 8 post-infection MARCO −/− mice had 71% smaller skin lesions than WT controls ( Fig. 5f , P <0.01, two-way analysis of variance). Together, these findings indicate that the interaction of HSV-1 gC and MARCO is functionally significant in HSV-1 infection and is relevant to cutaneous HSV-1 disease. We demonstrate using several independent lines of evidence that HSV-1 enhances adsorption and infection of keratinocytes by binding the scavenger receptor MARCO. Observations supporting this conclusion include competition experiments showing that the scavenger receptor ligand Poly(I) inhibited adsorption and infection of HSV-1 in cultured keratinocytes, inhibited purified gC binding to the cell surface, and inhibited HSV-1 infection in mouse skin. Furthermore, proximity ligation unambiguously detected the physical co-localization of HSV-1 gC and MARCO on cells, and analysis of binding showed direct high-affinity binding between MARCO and gC in cell free systems. Finally, overexpression of MARCO in keratinocytes increased susceptibility to infection while MARCO −/− mice were less susceptible to infection by HSV-1. Taken together, these findings show for the first time that MARCO expression on keratinocytes contributes to early infectious steps of HSV-1 in skin. Our results demonstrate that HSV-1 adsorption to keratinocytes involves more than just an interaction with HSPGs. We confirmed the previously reported [1] role of HSPGs in adsorption of HSV-1 as heparin was able to suppress gC binding and HSV-1 infection of keratinocytes. Syndecan-1, an HSPG that is highly expressed on the surface of keratinocytes, co-localized with gC and is the likely candidate for the HSPG to which gC binds. However, although previous studies have shown that HSV-1 infection can still occur in the absence of any cell surface HSPGs [46] , it was entirely unsuspected that the virus could usurp a scavenger receptor to promote adsorption. We have now demonstrated that gC co-localizes with MARCO and HSPGs on the cell surface, and gC bound directly to MARCO in the absence of other cellular or viral proteins. Interestingly, the affinity of gC to MARCO appeared to be measurably higher than the previously known binding affinity of gC to heparan sulphate. Furthermore, gC used distinct domains to bind to HSPGs and MARCO, because deletion of the C5/P (heparin binding) domain dramatically reduced gC binding to heparin but not to MARCO, and a mutant virus lacking the heparin-binding domain remained susceptible to inhibition by Poly(I). Previously, both Dxs and Fn were reported to be inhibitors of HSV-1 infection [47] . It was assumed that these compounds inhibited infection by preventing interaction of HSV-1 with HSPGs, however, both compounds had substantially lower minimum inhibitory concentrations than heparin, and it was not suspected that Dxs or Fn might also have acted against HSV-1 by competition with MARCO. Our results now suggest that the potent inhibitory of effects of these compounds may result from their capacity to block interactions with both HSPGs and MARCO. Thus, multiple lines of evidence show low affinity, high abundance (HSPGs) and high affinity, low abundance (MARCO) receptors are binding to gC and acting together to mediate adsorption and infection of keratinocytes. Beyond promoting adsorption and infection, the interaction with MARCO may also benefit HSV-1 by potentially enabling it to limit and evade innate immune responses. The binding of HSV-1 to MARCO may interfere with the function of MARCO to endocytose nucleic acids, thereby limiting the ability of cells to respond to exogenous nucleic acids via intracellular innate immune receptors like TLR3. Additionally, a recent study has indeed shown that although MARCO increases intracellular TLR recognition of nucleic acids, the presence of these receptors actually has the opposite effect on the ability of cell-surface TLRs to detect pathogens [48] . Thus, the interaction of HSV-1 with MARCO may increase adsorption and also limit cell-surface recognition of viral components by alternative innate immune receptors such as TLR2, which is also involved in the detection of HSV-1 (ref. 49 ). Further studies will be needed to evaluate the full consequences of the interaction of HSV-1 with MARCO. From a clinical standpoint, the protection conferred against HSV-1 infection by scavenger receptor ligands, and the significant reduction in infection in MARCO −/− mice, validated the physiological relevance of our observations. Although the role of gC in viral attachment in vitro has been well established, the complete virulence mechanism of gC in vivo is more complex than this binding interaction. Ultimate virulence involves several factors such as complement and antibody evasion, not only attachment [50] . The mouse model system used here employed scarification as a method to increase access to keratinocytes and to enhance local infection and amplification of the virus before spread to sensory ganglia [51] . These results showed in vivo that access to MARCO is required for optimal infection in the skin. However, it is not clear what role MARCO has in infection of other tissues. The efficacy of Poly(I) to inhibit HSV-1 infection in vivo was less than the effect seen on isolated keratinocytes in in vitro, and the reduction seen in MARCO −/− mice was not absolute. Further studies are needed to optimize treatment conditions to specifically block the multiple modes by which HSV-1 adsorbs to keratinocytes. Such therapies can be especially useful in diseases such as atopic dermatitis where epidermal susceptibility to viral infections is enhanced. Previous studies have shown that there are redundancies in the affinity and function of scavenger receptors in nucleic acid uptake [14] , [15] , and the role of other scavenger receptors in HSV-1 infection is not clear. Using a different route of infection (intravenous), Suzuki et al. [52] previously reported that MSR1 knockout mice were more susceptible to HSV-1 infection compared with WT mice. This raises the important possibility that the role of scavenger receptors might be specific to the route of administration, the type of receptor, and the cell target. As the subsequent recognition of viral nucleic acids by scavenger receptors is necessary for the later interferon response, it is possible that the observations with MSR1-deficient mice highlight the later immune defense role of this molecule. Future studies will be needed to fully understand the outcome of the interaction of HSV-1 with scavenger receptors and determine if these interactions are ultimately beneficial for the host or the virus. Some additional viruses have been previously suggested to interact with class A scavenger receptors. For example, MSR1 has been shown to be essential to the sensing of human cytomegalovirus by endosomal TLRs [17] , indicating a protective role for MSR1 in this context. In contrast, Adenovirus type 5 (ref. 53 ) has been recently shown to use MSR1 to facilitate infection. Additionally, it has been recently demonstrated that the presence of MARCO increases susceptibility to influenza, although MARCO does not enhance viral uptake and instead appears to suppress a beneficial early inflammatory response in the lungs [54] . Combined with our current study, these results emphasize the nuanced relationship existing between class A scavenger receptors and viruses. To our knowledge, this is the first demonstration that HSV-1 can utilize a component of the pattern recognition system to enhance disease. Our studies concur with other examples of HSV-1 modulating innate and adaptive immune systems to enhance virulence, but conflict with the current common understanding of epithelial immune defense systems that predicts that these elements are beneficial to the host [55] , [56] , or that association with viral recognition systems leads to protection against infection [57] , [58] . Exploitation of the cell surface scavenger receptor system by HSV-1 further illuminates the complexity of the interactions between the host and pathogen at the epithelial surface. Cells and animals and viruses NHEK (Life Technologies, Grand Island, NY) were cultured in Epilife media containing Epilife Defined Growth Supplement (Life Technologies, Grand Island, NY), 0.06 mM calcium chloride, and 100 IU Penicillin and 100 μg Streptomycin per ml (VWR, Radnor, PA). BSC-1 cells (ATCC, Manassas, VA) and HaCat keratinocytes (a gift from Rivkah Isseroff, University of California, Davis) were cultured in DMEM (Lonza, Basel, Switzerland), 10% FBS (Thermo Fisher Scientific, Waltham, MA), 2 mM L -glutamine and 100 IU Penicillin and 100 μg Streptomycin per ml (VWR, Radnor, PA). HaCat cells stably overexpressing MARCO and control HaCat cells were generated by transfecting HaCats with a pcDNA3 control plasmid or pcDNA3[MARCO], using the Nucleofector kit V and Nucleofector device (Lonza, Basel, Switzerland). Cells were cultured for 3 weeks in media containing 500 μg ml −1 G418 (Biopioneer, San Diego, CA) to select for transfected cells before use in experiments. These cells were continuously cultured in 500 μg ml −1 G418 during experiments. C57Bl/6 wild-type mice were purchased from the Jackson Laboratory, Bar Harbour, Maine. MARCO −/− mice were a gift from Dr Andrij Holian (Univerity of Montana, MT). All animal studies were in accordance with the Public Health Service Policy on Humane Care and Use of Laboratory Animals, and were approved by UCSD IACUC (UCSD Animal Welfare Assurance # A3033-1). All procedures were performed under isofluorane anaesthesia, and all efforts were made to minimize pain, discomfort and suffering. The NS strain of HSV-1 ( Fig. 1c , and Fig. 5c ), the gCΔC5/P mutant ( Fig. 1f ), and the gC Null mutant ( Fig. 5c ) were a generous gift from Dr Harvey Friedman (University of Pennsylvania, PA). The Schooler strain of HSV-1 was a generous gift from Dr William Fenical (Scripps Institute of Oceanography, CA). Plasmids A plasmid with a pcDNA3 backbone, expressing full-length human MARCO driven by a cytomegalovirus promoter, and a Neomycin resistance gene, pcDNA3[MARCO] (a gift from Sanjunkta Ghosh, Harvard University, Boston MA) was used for transfection experiments, with pcDNA3.1(-) (Life Technologies, Grand Island, NY) as a negative control plasmid. Reagents and primary antibodies Poly(I:C) was purchased from Invivogen, San Diego, CA. Poly(I), Poly(C), Dxs, Fn, CS, heparin, cyclophosphamide and methylthioadenosine was purchased from Sigma-Aldrich, St. Louis, MO. Chloroquine phosphate was purchased from Spectrum, Gardena, CA. Recombinant OLR1 was purchased from R&D Systems, Minneapolis, MN. Purified HSV-1 gC (gC1(457t)), gB (gB1(730)) and gC(Δ33-123t) (lacking the ΔC5/P domain) were generous gifts from Dr. Roselyn Eisenberg and Dr. Gary Cohen (University of Pennsylvania, PA). A cell line for the production of recombinant MARCO was kindly provided by Dr. Andrij Holian (Univerity of Montana, MT). MARCO protein was produced and purified as described [59] . Primary antibodies recognizing HSV-1 gC (mouse monoclonal, clone T96, catalogue no. sc-51626), HSV-1 gB (mouse monoclonal, clone 10B7, catalogue no. sc56987), MARCO (rabbit polyclonal, catalogue no. sc-68913), OLR1 (rabbit polyclonal, catalogue no. sc20753) and all IgG controls were purchased from Santa Cruz Biotechnology, Santa Cruz, CA. A monoclonal primary antibody recognizing HSV-1 gD (clone 2C10, catalogue no. ab6507) was purchased from Abcam, Cambridge, MA. A primary antibody recognizing Syndecan-1 was previously characterized [6] . A rabbit polyclonal antibody recognizing human SCARA3 (catalogue no. SAB2700220) was purchased from Sigma-Aldrich, St. Louis, MO. A mouse monoclonal antibody recognizing human MARCO was previously characterized [60] . A rat monoclonal antibody recognizing mouse MARCO (clone ED31, catalogue no. MCA1849) was purchased from Hycult Biotech, Plymouth Meeting, PA. A monoclonal antibody recognizing human glyceraldehyde 3-phosphate dehydrogenase (GAPDH) (clone 6C5, catalogue no. 10R-G109a) was purchased from Fitzgerald, Acton, MA. Fluorescence microscopy Cells were fixed with paraformaldehyde and blocked with 3% bovine serum albumin (Sigma-Aldrich, St. Louis, MO). Prolong 4',6-diamidino-2-phenylindole anti-fade and fluorescent Alexa Fluor conjugated secondary antibodies (1:200 dilution) were used (Life Technologies, Grand Island, NY). Images were captured using a BX41 microscope (Olympus, Center Valley, PA). Plaque assay Keratinocytes were infected with HSV-1 for 2 h, then washed and incubated in fresh media for 48 h. Cells were fixed and plaque formation visualized by staining cells with the anti-gD antibody (1:1 000), and an IR-Dye conjugated secondary antibody (1:10 000) (LI-COR Biosciences, Lincoln, NE) and imaging stained plaques using an Odyssey Imager (LI-COR Biosciences, Lincoln, NE). Multiplicity of infections selected resulted in ~100–200 plaques per well in a six-well plate using WT HSV-1, NS strain. Quantitative real-time PCR RNA and DNA were isolated using Trizol (Life Technologies, Grand Island, NY). RNA was reverse transcribed using iScript (Bio-Rad, Hercules, CA). Predesigned Taqman probes and primers were used to quantify IL-6, IL-8, human beta-defensin 2 and IFN-β messenger RNA using Taqman Gene Expression Master Mix and a 7300 Real Time PCR System (Life Technologies, Grand Island, NY) according to the manufacturer’s instructions. Custom Taqman Probes (Life Technologies, Grand Island, NY) were used for HSV-1 gD and GAPDH RNA and DNA quantification. HSV-1 gD probe: FAM-CCATACCGACCACACCGACGAACC-MGB; GAPDH probe: VIC-CATCCATGACAACTTTGG TA-MGB. Primers sequences (Sigma-Aldrich, St Louis, MO): HSV-1: 5′-CGGCCGTGTGACACTATCG-3′, 5′-CTCGTAAAATGGCCCCTCC-3′; GAPDH: 5′-CCTAGCACCCCTGGCCAAG-3′, 5′-TGGTCATGAGTCCTTCCACG-3′. Fold change normalized to host cell GAPDH levels relative to the control was calculated using the 2 (−ΔΔCt) method. Enzyme-linked immunosorbent assay IL-6 concentration was determined using an OptEIA enzyme-linked immunosorbent assay (ELISA) Set (BD Biosciences Pharmigen, San Diego, CA). HSV-1 immunofluorescence adsorption assay HSV-1 was incubated with cells at 4 °C for 2 h, then cells were washed to remove unbound virus, fixed with paraformaldehyde and stained using an HSV-1 gC antibody (1:100), and an Alexa-Fluor labelled secondary antibody (1:200) (Life Technologies, Grand Island, NY). Images were taken by fluorescent microscopy (described above) and HSV-1 particles were quantified using ImageJ. The specificity of this assay was validated by control experiments using serial diluted HSV-1. Western blot Protein was isolated by lysing cells at 4 °C in 1 × RIPA buffer containing protease inhibitors (Roche, Basel, Switzerland) and protein concentrations quantified using a BCA assay (Thermo Fisher Scientific, Waltham, MA). Twenty microgram total protein was loaded on a 4–20% agarose gel and transferred to a polyvinylidene difluoride (membrane Bio-Rad, Hercules, CA). MARCO protein was detected using the rabbit polyclonal antibody (1:1 000) and GAPDH was detected using the mouse monoclonal antibody (1:10 000). Six-hundred and eighty nanometre and 800 nm IR-Dye conjugated secondary antibodies (1:10 000) and an Odyssey imager and quantification software (LI-COR Biosciences, Lincoln, NE) were used for two-colour western blotting to analyse both proteins on the same blot. On-cell western gC cell-binding assay gC was incubated with cells and the indicated compounds together at 4 °C. Cells were washed before fixation. Bound gC was detected with the anti-gC antibody (1:100) and an IR-Dye conjugated secondary antibody (1:800) (LI-COR Biosciences, Lincoln, NE), and an Odyssey imager (LI-COR Biosciences, Lincoln, NE). A standard curve was generated using serial dilutions of known concentrations of gC bound to cells to quantify the amount of bound gC. ELISA-binding assay Capture protein was bound to EIA/RIA plates (Thermo Fisher Scientific, Waltham, MA) in PBS lacking calcium and magnesium, pH 7.4 (Life Technologies, Grand Island, NY), blocked with PBS containing 3% BSA (Sigma-Aldrich, St. Louis, MO), then incubated with viral glycoproteins diluted in PBS. Cells were washed with PBS containing 0.05% Tween-20. Bound glycoproteins were detected using primary antibodies (1:200), horseradish peroxidase-conjugated secondary antibodies (1:500) (Santa Cruz Biotechnology, Santa Cruz, CA), and 3,3′, 5,5′-tetramethylbenzidine substrate reagent (BD Biosciences Pharmigen, San Diego, CA). Standard curves for quantification of bound viral glycoproteins were generated using serial dilutions of known concentrations of the proteins. High-performance liquid chromatography A HiTrap Heparin HP Column and AKTA purifier high-performance liquid chromatography (HPLC) system (GE Healthcare, Piscataway, NJ) were used for analysis. Briefly, 100 μg of purified gC protein was loaded on to the heparin column and the column was washed to remove any unbound gC. Freshly prepared Poly(I) and NaCl solutions were used to generate the indicated concentration gradients used for elution. One millilitre fractions were collected during the elution, and the amount of gC present in these fractions was quantified by dot blot using the anti-gC antibody (1:1 000), an IR-Dye conjugated secondary antibodies (1:10 000) (LI-COR Biosciences, Lincoln, NE), and an Odyssey imager (LI-COR Biosciences, Lincoln, NE) with known concentrations of purified gC protein used to generate a standard curve for quantification. HSV-1 infection of immunocompromised mice Mice were injected intraperitoneally with 300 mg kg −1 cyclophosphamide. One day later, mice were depilated. Two days after cyclophosphamide injection, mice were infected with 10 5 PFU HSV-1 by scarification with 25G needles. Mice were photographed once daily, and lesion sizes were quantified using ImageJ. Mice were euthanized when they became extremely lethargic and/or exhibited signs of paralysis, indicating systemic spread of the virus and imminent mortality. Proximity ligation assay NHEK seeded into chamberslides (Thermo Fisher Scientific, Waltham, MA) were incubated with HSV-1 or gC for 2 h at 4 °C allowing binding, but not internalization. Unbound virus or protein was removed by washing with cold PBS. Cells were fixed with paraformaldehyde at 4 °C. Blocking buffer (O-link Bioscience, Uppsala, Sweden) was used to prevent nonspecific antibody binding, and cells were incubated with two primary antibodies (1 μg ml −1 ), one recognizing gC and the other recognizing the indicated proteins, MARCO, Syndecan-1, OLR1 and SCARA3. Secondary antibodies conjugated with oligonucleotides were added, and hybridization, ligation, amplification and detection steps were performed according to the manufacturer’s instructions (O-link Bioscience, Uppsala, Sweden) to generate an amplified fluorescent signal in areas where the antigens recognized by the two primary antibodies reside within less than ~40 nm. Fluorescent PLA signals were evaluated using fluorescence microscopy (described above). Statistical analysis Analyses were performed using GraphPad Prism version 5.00 for Windows, GraphPad Software, San Diego, California, USA, www.graphpad.com . How to cite this article: MacLeod, D. T. et al. HSV-1 exploits the innate immune scavenger receptor MARCO to enhance epithelial adsorption and infection. Nat. Commun. 4:1963 doi: 10.1038/ncomms2963 (2013).